Realization of a spin-wave multiplexer Recent developments in the field of spin dynamics—like the interaction of charge and heat currents with magnons, the quasi-particles of spin waves—opens the perspective for novel information processing concepts and potential applications purely based on magnons without the need of charge transport. The challenges related to the realization of advanced concepts are the spin-wave transport in two-dimensional structures and the transfer of existing demonstrators to the micro- or even nanoscale. Here we present the experimental realization of a microstructured spin-wave multiplexer as a fundamental building block of a magnon-based logic. Our concept relies on the generation of local Oersted fields to control the magnetization configuration as well as the spin-wave dispersion relation to steer the spin-wave propagation in a Y-shaped structure. Thus, the present work illustrates unique features of magnonic transport as well as their possible utilization for potential technical applications. Recently, several new concepts were presented that associated with a novel magnonic approach for information transport and processing [1] , [2] , [3] , [4] , [5] , [6] , [7] . Magnons are the spin-wave excitation quanta of magnetic materials. They can be understood classically as the collective precession of the electrons’ spins. The collective nature is mediated by the short-range quantum–mechanical exchange interaction, as well as the non-local magnetic dipole interaction. Spin waves carry spin angular momentum, as do electrons in spintronic applications [8] , [9] , and enable the coherent transport of information encoded in its phase and amplitude. However, in contrast to spin-polarized electron-based spintronics, spin waves do not require dissipative charge transport that is subject to unavoidable scattering of individual electrons. Spin waves are collective excitations of the electronic system and propagate over significantly larger distances compared with typical electron spin diffusion lengths in metals or semiconductors, even at room temperature. Typical loss channels for spin waves, for example, spin–orbit interaction, can be minimized by the choice of suitable materials like yttrium iron garnets [10] or Heusler compounds [11] , [12] . Furthermore, spin waves have the advantage that their frequencies increase faster for decreasing feature sizes in comparison to electromagnetic waves. Thus, even at 0.1–1 THz, spin-wave wavelengths can be as short as only a few nanometres, which is orders of magnitudes smaller compared with electromagnetic waves. This facilitates higher integration density in spin-wave logic devices. Spin waves exhibit a peculiarity that differentiates them from light or sound waves: their dispersion relation is highly anisotropic [13] , [14] . This means that their energy significantly depends on the relative angle between their propagation direction and the magnetization orientation. As a result, if the magnetic material is exposed to a uniform external magnetic field, the spin waves will travel in the preferred direction with respect to the magnetization orientation. The need for such external magnetic fields has hampered the development of spin-wave devices that are based on combining spin waves in two dimensions. Thus, even though simulations of nanometre-sized Mach–Zehnder-type interferometers demonstrate the feasibility to build spin-wave logic gates [15] , [16] , their realization to date has only been accomplished on the millimetre scale [17] . Herein we demonstrate a simple implementation of a microstructured spin-wave multiplexer, which serves as an initial step towards the development of a viable spin-wave-based processor. In our approach, locally generated magnetic fields, rather than uniform external fields, alter the magnetization direction solely in designated regions of the spin-wave multiplexer. This enables us to tailor the dispersion relation in different parts of the structure to our advantage [18] . Thereby, we exploit the unique feature of the anisotropic dispersion relation of spin waves, and, thus, are able to switch spin-wave propagation directions. 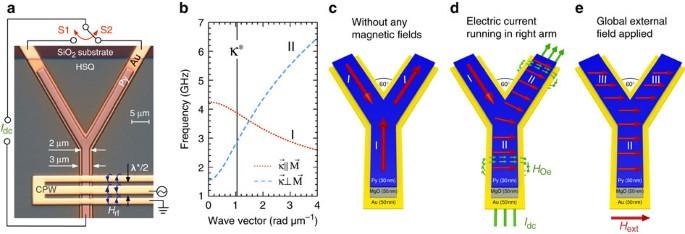Figure 1: Sample layout, spin-wave dispersions and magnetic ground states. (a) Microscope image showing the spin-wave multiplexer, the microwave antenna (CPW: coplanar waveguide) and the leads for direct current connections. Blue arrows indicate the oscillating Oersted fieldsaround the antenna. (b) Dispersion relations for parallel (dotted line) and perpendicular (dashed line) alignment of the spin-wave wave vectorand the magnetization, corresponding to regions I and II in the schematics of the magnetization distribution. The fieldμ0HOe=10.3 mT used for the dispersion calculation in region II corresponds to a current ofIdc=100 mA in the gold layer. This current was used in the measurements presented below. The dispersion calculation for region I corresponds to zero field. Schematics of the magnetization configurations in remanence (c), with locally generated Oersted field (d) and with an externally applied magnetic field (e). Sample characteristics and concept Figure 1a shows an optical microscope image of the device. Using electron-beam lithography and lift-off techniques, a 30-nm-thick Ni 81 Fe 19 (permalloy, Py) layer was patterned into a Y-shaped spin-wave waveguide having a constant width of 2 μm. To evaluate a possible angle dependence of the spin-wave propagation, structures with the opening angles 30°, 60° and 90° were fabricated and tested experimentally. In the following we will concentrate on the 60° structure where the best results were obtained. A comparison of the different structures will be presented later in the article. Figure 1: Sample layout, spin-wave dispersions and magnetic ground states. ( a ) Microscope image showing the spin-wave multiplexer, the microwave antenna (CPW: coplanar waveguide) and the leads for direct current connections. Blue arrows indicate the oscillating Oersted fields around the antenna. ( b ) Dispersion relations for parallel (dotted line) and perpendicular (dashed line) alignment of the spin-wave wave vector and the magnetization , corresponding to regions I and II in the schematics of the magnetization distribution. The field μ 0 H Oe =10.3 mT used for the dispersion calculation in region II corresponds to a current of I dc =100 mA in the gold layer. This current was used in the measurements presented below. The dispersion calculation for region I corresponds to zero field. Schematics of the magnetization configurations in remanence ( c ), with locally generated Oersted field ( d ) and with an externally applied magnetic field ( e ). Full size image To control the magnetization direction in the Y structure with local Oersted fields, a 50-nm thick and 3-μm wide Au conduit was fabricated below the spin-wave waveguide. Leads at the three ends of the Au conduit allow for connecting either its base and left arm (switch in Fig. 1a in position S1) or its base and right arm (switch in position S2) to an electric current source, respectively. To keep the electric current from flowing in the magnetic material, a 50-nm thick MgO layer serves as an insulator from the Au conduit. A microwave current in the shorted coplanar waveguide generates oscillating magnetic fields that excite spin waves in the Py waveguide. For in-plane magnetized films, the anisotropic dispersion relation favours propagation perpendicular to the magnetization direction . As depicted by the dispersion relations [19] in Fig. 1b (calculated with the material parameters for Ni 81 Fe 19 : saturation magnetization: M S =800 kA m −1 , gyromagnetic ratio: γ /2π=28 GHz T −1 and exchange constant: A =1.6 × 10 −11 J m −1 ), a perpendicular orientation between the spin-wave wave vector and the magnetization direction (dashed, blue line, geometry II) results in a higher group velocity, which is given by the slope of the dispersion, compared with the case of parallel alignment (dotted, red line, geometry I). Thus, spin-wave transport perpendicular to suffers less spatial decay. The dispersion calculation for region II corresponds to an Oersted field of μ 0 H Oe =10.3 mT resulting from a current of I dc =100 mA in the Au conduit as used in all the measurements presented below. Without any applied magnetic fields, however, the shape anisotropy of the microstructured waveguide forces the magnetization to align along the spin-wave waveguide, as is depicted in Fig. 1c , since magnetic moments pointing transverse to the waveguide give rise to energetically unfavourable magnetic surface charges. In the absence of additional magnetic anisotropies, the energy that is required to maintain a transverse magnetization needs to be provided by an external magnetic field. In the spin-wave multiplexer presented here, local Oersted fields are induced by the electric current flowing in the Au conduit. As a consequence, the magnetization configuration inside the Y-shaped microstructure can be controlled in several ways: without any external magnetic field and any direct current in the Au conduits, is in remanence and aligns along the boundaries of the waveguide, as shown in Fig. 1c . If a direct current I dc runs in the base and the right arm of the Y structure, as is the case in Fig. 1d , only the magnetic moments in this region will be forced to point transverse to the waveguide. Consequently, a spin wave that is excited in the base of the Y structure will propagate along the path that provides an undisturbed magnetization configuration, that is, into the right arm. In addition to the higher group velocity that favours propagation in the right arm, the field inhomogeneity caused by the domain wall at the intersection of the base and the left arm acts as a potential barrier and, thus, hinders propagation in the left arm. If a uniform external magnetic field is applied, the magnetic moments of the Ni 81 Fe 19 will be aligned along the direction of this field, as illustrated in Fig. 1e . Consequently, the angle between and the spin-wave wave vector will change in the transition between the base and both arms, prohibiting spin-wave propagation beyond the junction of the Y structure, as we show below. Experimental demonstration To evaluate the functionality of the proposed spin-wave multiplexer, we employed Brillouin light scattering (BLS) microscopy [20] , [21] . Measuring the BLS intensity for various excitation frequencies inside the arms of the Y-shaped multiplexer enables us to determine whether the spin-wave propagation path can be switched. In Fig. 2a , 100-mA current pulses were applied to the right arm only. For excitation frequencies ranging from 2 to 4 GHz, we then recorded the spin-wave intensity 4.5 μm behind the Y junction in the right (red circles) and left arm (blue squares). As can be seen, spin waves are solely detected inside the right arm where the magnetization is forced to the preferred propagation geometry II by the local Oersted fields (compare Fig. 1d ). The measurement inside the left arm does not yield a spin-wave signal. The situation is reversed if the electric current is flowing in the left arm of the Au conduit, as is shown in Fig. 2b . Only the measurement in the left arm shows a spin-wave signal (blue squares). This confirms the functionality of the spin-wave multiplexer. Using the electric current, we are able to switch the spin-wave propagation direction between the two arms of the Y-shaped waveguide. 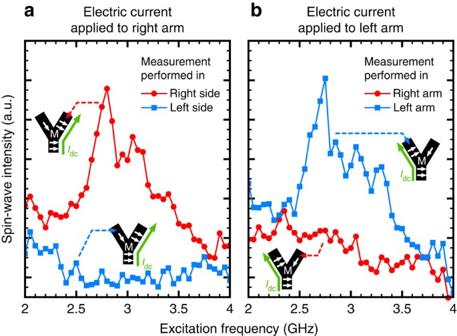Figure 2: Spin-wave transmission spectra. Spin-wave intensities measured for excitation frequencies ranging from 2 to 4 GHz and an electric current of 100 mA flowing in the right (a) and left (b) arms of the Y structure. For both magnetization configurations, red circles denote the spin-wave intensity inside the right arm, whereas blue squares denote the intensity inside the left arm, both measured at 4.5 μm distance from the Y junction. Figure 2: Spin-wave transmission spectra. Spin-wave intensities measured for excitation frequencies ranging from 2 to 4 GHz and an electric current of 100 mA flowing in the right ( a ) and left ( b ) arms of the Y structure. For both magnetization configurations, red circles denote the spin-wave intensity inside the right arm, whereas blue squares denote the intensity inside the left arm, both measured at 4.5 μm distance from the Y junction. Full size image A closer look at Fig. 2 reveals that only spin waves in the frequency range between 2.5 and 3.4 GHz propagate beyond the junction of the multiplexer. This is related to the spin-wave dispersion relation as well as to the excitation efficiency of the antenna. The small blue arrows in Fig. 1a illustrate the oscillating magnetic fields generated by the coplanar waveguide. Its periodicity imposes a wavelength of λ *=6 μm and, thus, a wave vector of k *=1.05 rad μm −1 for which spin waves are excited most efficiently. As can be seen from the dashed dispersion relation in Fig. 1b , this wave vector corresponds to a frequency of 2.75 GHz, matching the frequency for which the spin-wave intensities detected in Fig. 2 reach their maxima. For lower and higher frequencies, the excitation efficiency of the antenna drops drastically. In addition, evaluating the slope of the dispersion relation shows that the group velocity is largest for the same spin-wave frequency of 2.75 GHz. Consequently, spin waves excited at this frequency propagate a longer distance before they attenuate and, thus, can be detected inside the arms. Ultimate evidence for the functionality of the spin-wave multiplexer is obtained from the measured two-dimensional spin-wave intensity distributions. For the switching experiment, the excitation frequency of 2.75 GHz was chosen to match the maximum intensity that was previously determined inside the arms (see Fig. 2 ). 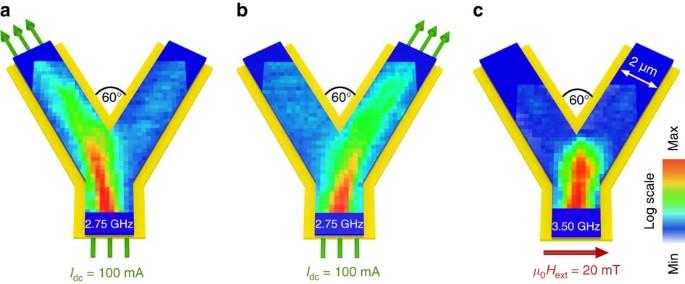Figure 3: Proof of spin-wave switching. Two-dimensional mapping of the spin-wave propagation path illustrating the switching: For a direct current of 100 mA applied to the left (a) and right (b) arms of the Y structure, the spin waves at 2.75 GHz are guided through the Y junction and only propagate in the same direction as the current flow. (c) Saturation with an external magnetic fieldobscures any spin-wave transport beyond the junction. Figure 3a illustrates the case for current pulses with 100 mA amplitude flowing in the left arm of the Au conduit. The spin-wave intensity scale is logarithmic and colour coded, where red (white) represents the maximum (minimum) intensity. It is obvious that with the current flowing in the left pathway, the spin wave reaches the bifurcation and turns into the left arm only. Inside the right arm, no spin-wave intensity can be detected. When the 100-mA current pulses are applied to the right arm, as is the case in Fig. 3b , the spin wave only propagates into the right arm. This illustrates the possibility to switch the information channel in the proposed spin-wave multiplexer by means of locally generated Oersted fields. Surprisingly, Fig. 3c shows that spin-wave propagation is entirely prohibited behind the Y junction in case a uniform external magnetic field is applied. Spin waves are known to adiabatically adjust their wavelength in regions of inhomogeneous magnetic field strengths to compensate for magnetic field-induced shifts of the dispersion [22] , [23] . However, apparently, spin-wave transport is prohibited if the relative orientation between the magnetization direction and the spin-wave wave vector changes. This provides new ways to manipulate spin-wave transport in magnetic microstructures. Figure 3: Proof of spin-wave switching. Two-dimensional mapping of the spin-wave propagation path illustrating the switching: For a direct current of 100 mA applied to the left ( a ) and right ( b ) arms of the Y structure, the spin waves at 2.75 GHz are guided through the Y junction and only propagate in the same direction as the current flow. ( c ) Saturation with an external magnetic field obscures any spin-wave transport beyond the junction. Full size image As already pointed out, additional structures with the alternative opening angles of 30° and 90° were also investigated to test the angle dependence of the spin-wave switching. A comparison between the different structures is illustrated in Fig. 4 . As can be seen, the Y structure with the opening angle of 60°, which was used for the measurements presented above, yielded the largest propagation distance along the current path and, thus, the best conditions for the spin-wave switching. 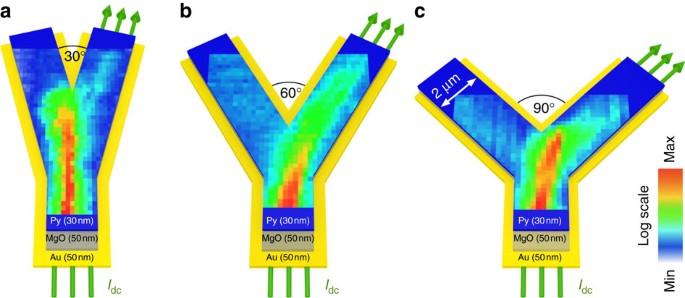Figure 4: Angle dependence of the spin-wave switching. Propagation of spin waves through spin-wave multiplexers with different opening angles: (a) 30°, (b) 60° and (c) 90°. A direct current of 100 mA was applied to the right arm of the Y structures. The excitation frequency was fixed to 2.75 GHz. Figure 4: Angle dependence of the spin-wave switching. Propagation of spin waves through spin-wave multiplexers with different opening angles: ( a ) 30°, ( b ) 60° and ( c ) 90°. A direct current of 100 mA was applied to the right arm of the Y structures. The excitation frequency was fixed to 2.75 GHz. Full size image The varying performance of the devices can be understood as follows. For the 30° structure, the intersection of the base and the two arms occupies a larger area than in the case of larger opening angles. This increased area leads to a decrease in the current density and, thus, in the corresponding Oersted field. As a result, the propagation distance of spin waves following the current path drops. For the large opening angle of 90°, a very abrupt change of the spin-wave wave vector is needed to adjust to the new propagation direction. As indicated by our results, this leads to decreased propagation in the right arm. The intermediate angle of 60° is a reasonable trade-off between a strongly varying current density at the intersection between base and arm and a strong change in direction of waves propagating in one of the arms. These additional considerations have to be taken into account regarding the design of similar spin-wave devices as well as regarding two-dimensional spin-wave transport in general. In conclusion, we have demonstrated how the spin-wave propagation path can be manipulated in a prototype spin-wave multiplexer on the micrometre scale using locally generated magnetic fields. We want to emphasize that the dimensions of the devices discussed here were chosen to optimize the optical investigation of their operation. However, there are no physical limitations for miniaturizing them into the nanometre regime. Furthermore, the same approach can be adapted to ferromagnetic insulators, such as yttrium iron garnets, where the damping of the magnetization dynamics is greatly reduced and therefore the spin-wave propagation distance is significantly increased. Another approach to reduce the currents required to magnetize the spin-wave waveguide perpendicular to the transport direction is to use ion implantation to imprint waveguides into paramagnetic or ferromagnetic films [24] , [25] . In such waveguides the shape anisotropy is strongly reduced due to the surrounding ferro- or paramagnetic environment. Lastly, while we use Oersted fields to readily vary local magnetic fields, it is also conceivable to use switchable stray fields from adjacent magnetic elements [26] or direct exchange coupling [27] that would enable a low-power operation of the spin-wave multiplexer in more complex magnonic devices. Sample preparation The samples were prepared in four steps using electron-beam lithography, sputter-deposition in ultrahigh vacuum and subsequent lift-off processes to prepare the sample structure consisting of (1) the Au conduits for the application of the direct current pulses, (2) the Ni 81 Fe 19 spin-wave waveguide on top of an insulating MgO layer, (3) a hydrogen silsesquioxane (HSQ) layer to insulate the underlying layers electrically from (4) the Au microwave antenna. The large Au leads at the end of the current lines were prepared in a fifth step with optical lithography using a laser-writer system. Local Oersted fields and spin-wave excitation Local Oersted fields were created by the application of 100-mA current pulses to the Au leads. To avoid excessive heating, we applied current pulses with a duration of 150 ns and a repetition rate of 3 μs. The amplitude of the resulting Oersted field was determined via a simulation using the software CST Microwave Studio. Spin waves were excited by 100-ns long microwave pulses synchronized to the direct current pulses. BLS microscopy All measurements were performed at room temperature. The spin-wave intensity is locally recorded by means of BLS microscopy. This method is based on the inelastic scattering of photons and magnons. Light from a continuous wave, single-frequency 532-nm solid-state laser is focused on the sample surface using a high numerical aperture microscope lens giving a spatial resolution of 250 nm. The laser power on the sample surface is typically about 2–3 mW. The frequency shift of the inelastically scattered light is analysed using a six-pass Fabry Perot interferometer TFP-1 (JRS Scientific Instruments). To record two-dimensional maps of the spin-wave intensity distribution, the sample is moved via a high-precision translation stage (10-nm step size, Newport). The sample position is continuously monitored with a CCD camera using the same microscope lens. A home-built active stabilization algorithm based on picture recognition allows for controlling the sample position with respect to the laser focus with a precision better than 20 nm. How to cite this article: Vogt, K. et al. Realization of a spin-wave multiplexer. Nat. Commun. 5:3727 doi: 10.1038/ncomms4727 (2014).